Suppression of the intrinsic stochastic pinning of domain walls in magnetic nanostripes Nanofabrication has allowed the development of new concepts such as magnetic logic and race-track memory, both of which are based on the displacement of magnetic domain walls on magnetic nanostripes. One of the issues that has to be solved before devices can meet the market demands is the stochastic behaviour of the domain wall movement in magnetic nanostripes. Here we show that the stochastic nature of the domain wall motion in permalloy nanostripes can be suppressed at very low fields (0.6–2.7 Oe). We also find different field regimes for this stochastic motion that match well with the domain wall propagation modes. The highest pinning probability is found around the precessional mode and, interestingly, it does not depend on the external field in this regime. These results constitute an experimental evidence of the intrinsic nature of the stochastic pinning of domain walls in soft magnetic nanostripes. The demand for higher areal densities on magnetic memories led to the introduction of novel concepts such as the Race-track memory [1] . This memory functions by moving the bits of information themselves (magnetic domains) rather than by spinning the disc under the reading head. Each magnetic domain is separated by a magnetic domain wall (DW) that can be moved with an external magnetic field or with a spin polarized current, being the second option the one with real interest for practical applications. Understandably, in a future commercial device, the DW would have to move reliably between engineered pinning sites millions of times, without ever getting stuck on the inevitable structural defects (crystalline defects, grain texture, edge roughness, etc). For other applications like magnetic logic [2] , or radio-frequency generation by the oscillation of a DW, the exact position of the DW must also be achieved and determined very reliably. It is well known that, in macroscopic magnetic elements, the DW travels in small discontinuous steps known as Barkhausen jumps, caused by the pinning and subsequent release of the DW from the defects in the materials. Similarly, in magnetic nanostripes (the basic constituent of the above-mentioned applications), the DW motion is also troubled by defects [3] , [4] . Low anisotropy materials like Permalloy (Ni 80 Fe 20 ) are generally used to study the DW motion in magnetic nanostripes, although materials with perpendicular-to-plane anisotropy are also attractive because the polarized current can be more effective at moving the DW. Both types of materials suffer from uncontrolled DW pinning [5] , [6] and, especially in the case of materials with perpendicular-to-plane anisotropy, even time-dependent thermal depinning. Recent studies on DW pinning on notch-free Permalloy nanostripes [4] , [7] , [8] have highlighted the stochastic nature of the DW motion. Whether the DW pinning is avoidable or intrinsic to the propagation of DWs in real nanostripes is a matter of debate and concern. Here we show that the DW stochastic pinning follows three different field regimes that match the DW propagation modes, indicating that it might indeed be intrinsic to the nature of the DW motion in nanostripes. On the other hand, we also show that the stochasticity of the DW pinning can be suppressed at very low fields and the DW transmission in a soft Permalloy nanostripe can be perfectly reliable. Interestingly, the pinning probability reaches its maximum value at intermediate fields (10–35 Oe) and it is constant (independent of the external field) in this range of fields. Pinning probability and efficiency of DW injection This study has been done on several Permalloy nanostripes, all 10 nm thick and 300 nm wide. The stripe has two sections, one with a notch and the other without any (intentional) defect ( Fig. 1a ). A conductive current line is placed in the centre and perpendicular to the stripe. A current pulse flowing through this central contact (length from 5 to 100 ns) nucleates a pair of DW that, in the presence of a positive magnetic field, travel in opposite directions [9] . The presence of a DW on any of the sections of the stripe can be detected by the drop in resistance associated with its anisotropic magnetoresistance. 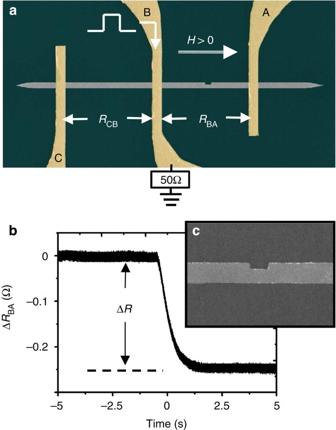Figure 1: Experimental set-up. (a) Coloured scanning electron microscopy picture of one of the nanostripes used in this work. The width of the stripe is 300 nm. A current pulse is introduced from contact B to ground, creating two magnetic domain walls that travel towards section AB (with a notch) and to section BC (without a notch). The direction of positive fields is indicated here. (b) The presence of the magnetic domain wall either in section AB or BC or both, is detected by the drop in the resistance of the stripe associated with the domain wall anisotropic mangetoresistance. (c) Zoom of the notch in section AB. The width of the stripe is 300 nm. Figure 1b shows the drop in resistance produced by the injection of a DW in section AB, when a current pulse is sent through the central current line. The integration time used to detect the resistance of the DW is 2 s, which is much longer than the time required for the DW to travel through the entire length of the nanostripe (tens of nanoseconds). Therefore, when a DW is detected by this method, it is at rest pinned somewhere along the stripe. Figure 1: Experimental set-up. ( a ) Coloured scanning electron microscopy picture of one of the nanostripes used in this work. The width of the stripe is 300 nm. A current pulse is introduced from contact B to ground, creating two magnetic domain walls that travel towards section AB (with a notch) and to section BC (without a notch). The direction of positive fields is indicated here. ( b ) The presence of the magnetic domain wall either in section AB or BC or both, is detected by the drop in the resistance of the stripe associated with the domain wall anisotropic mangetoresistance. ( c ) Zoom of the notch in section AB. The width of the stripe is 300 nm. Full size image The DW travelling to section AB is likely to get pinned at the notch. The detection of this DW allows us to be certain that the current pulse successfully injected a pair of DWs for a given pulse amplitude, and that one of them travelled through section BC. Note also that the pulse current only flows through the conductive current line and not through the magnetic nanostripe. Only the current used to measure the resistance of sections AB and BC flows through the nanostripe and it is too small to interfere with the movement of the DW by spin transfer (20 μA or 7×10 5 A cm −2 ). First, we analyse the efficiency of the current pulse to inject a pair of DW. 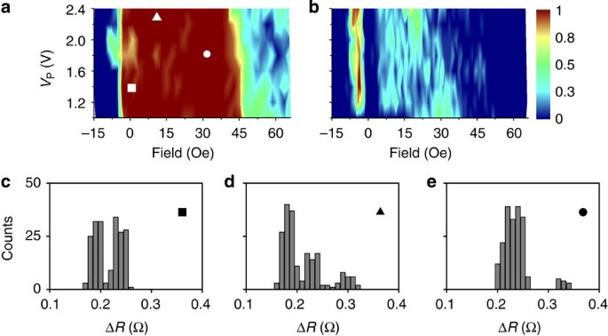Figure 2: Probability of pinning and type of magnetic domain wall. (a) Contour plot showing the probability of pinning a magnetic domain wall in section AB of the nanostripe pictured inFigure 1a, versus the voltage amplitudeVPof a 25 ns injection pulse (y-axis) and the external magnetic field (x-axis). The colour code for the probability is on the right. (b) Contour plot showing the probability of pinning a magnetic domain wall in the section BC of the nanostripe pictured inFigure 1a. (c–e) Histograms showing the resistance measured in every pinning event recorded for three different points of the probability map at section AB, 1.4 V–0 Oe inc, 2.4 V–10 Oe inband 1.8 V–35 Oe inc. These histograms show four different resistances 0.19, 0.23, 0.29 and 0.32 Ω, corresponding to different types of domain wall: Transversal with up and down symmetry and Vortex counterclockwise and clockwise, respectively. Figure 2a shows the probability of detecting a DW pinned at the notch (section AB) for a range of pulse amplitudes and magnetic fields. The conversion factor for the current pulse is 1.45×10 8 Acm −2 V −1 . As shown in Figure 2a , the probability of pinning a DW at the notch is 1 for all pulse amplitudes. Figure 2a gives an idea of how reliable the process of injection of a DW is. The resistance of the DW at each pinning event can be recorded, so we know the type of DW present in our stripes. The histograms at Figure 2c–e , show the four values of DW resistance in our stripes. The two lower values (0.19 and 0.23 Ω) correspond to transversal DW (TW) each of different symmetry and the two higher values (0.29 and 0.32 Ω) are vortex DW (VW) each of different chilarities [10] . Figure 2: Probability of pinning and type of magnetic domain wall. ( a ) Contour plot showing the probability of pinning a magnetic domain wall in section AB of the nanostripe pictured in Figure 1a , versus the voltage amplitude V P of a 25 ns injection pulse ( y -axis) and the external magnetic field ( x -axis). The colour code for the probability is on the right. ( b ) Contour plot showing the probability of pinning a magnetic domain wall in the section BC of the nanostripe pictured in Figure 1a . ( c – e ) Histograms showing the resistance measured in every pinning event recorded for three different points of the probability map at section AB, 1.4 V–0 Oe in c , 2.4 V–10 Oe in b and 1.8 V–35 Oe in c . These histograms show four different resistances 0.19, 0.23, 0.29 and 0.32 Ω, corresponding to different types of domain wall: Transversal with up and down symmetry and Vortex counterclockwise and clockwise, respectively. Full size image For a nanostripe without a notch, intuitively one might expect zero probability for pinning a DW. As can be seen from Figure 2b , this is far from true. The probability of pinning is 1 for slightly negative fields, then drops to zero for small positive fields and rises again to probabilities ranging from 0 to ∼ 0.5 before it finally drops to zero for fields larger than 50 Oe. This non-zero probability for the pinning of the DW on the section of the stripe without a notch could be put down to bad stripe quality, there being many fabrication defects that act as pinning sites. However, this cannot be the reason as there is a zone at low-positive fields where the probability of pinning is zero (that is, the DW travels through the stripe without ever pinning). Regimes of the pinning probability To better understand the behaviour of the DW travelling through a stripe without a notch, we have recorded the resistance at each pinning event. 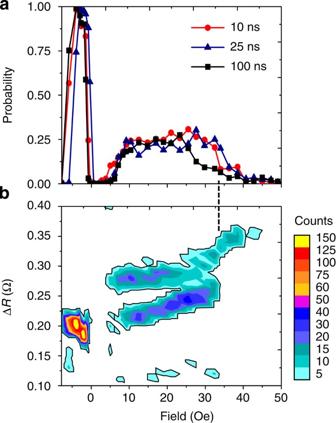Figure 3: Different regimes for the pinning probability. (a) Pinning probability (0–1) for the section BC of the nanostripe (calculated out of 400 injected domain walls for each magnetic field measured) versus the external magnetic field for different pulse lengths keeping the pulse amplitude constant in 1.4 V. (b) Contour plot made out of the histograms of resistivity for the pinning events (out of 400 injected domain walls for each field), for a 1.4 V–10 ns injection pulse (red curve ina). The black dashed line shows how the drop of the pinning probability in the red curve ona, corresponds with the disappearance of the low-resistive domain walls (Transversal domain wall). Note that the colour scale on the right is not linear. Figure 3a shows the probability of pinning for the section BC of the stripe for a 1.4 V pulse and different pulse lengths. Figure 3b shows the resistance map for all the pinning events for the case of a 1.4 V–10 ns injection pulse. Again in Figure 3a, we see very distinctive regimes, depending on the external magnetic field. For slightly negative fields, the probability is 1 and the type of DW is always transversal (Δ R =0.19 Ω). This is the region where the injected DW gets pinned just by the conductive current line that acts as a pinning site. Only for fields more negative than −8 Oe, the DW can pass underneath the current line and implode with the other DW. For positive magnetic fields from 0 to ∼ 3 Oe, the probability drops to zero, indicating that the DW is transmitted reliably through section BC of the stripe (the one without the notch). We have measured more than ten different nanostripes with the same dimensions, for different amplitudes of the injection pulse (from 1.2 to 2.4 V) and different lengths (from 5 to 100 ns). Taking into account all the measured devices, we have recorded the probability of pinning in the low -field range for many thousands of injection events (an 'event' is the successful injection of a DW, whether it gets pinned or not) and have not found a single pinning event in the range from 0.6 to 2.7 Oe. This shows that the stochastic propagation of a DW in a magnetic nanostripe can be totally suppressed at very low fields. This range of perfect reliability in the transmission probability can easily be missed in stripes of lower quality where the propagation field is 2 Oe, or more, as we ourselves have observed in some stripes with abnormally high-edge roughness or strong random defects. It can also be missed in experiments that use electrical current to induce the DW motion, where the critical current (minimum current necessary to achieve DW motion by spin transfer) might be equivalent to a higher field range [11] . Figure 3: Different regimes for the pinning probability. ( a ) Pinning probability (0–1) for the section BC of the nanostripe (calculated out of 400 injected domain walls for each magnetic field measured) versus the external magnetic field for different pulse lengths keeping the pulse amplitude constant in 1.4 V. ( b ) Contour plot made out of the histograms of resistivity for the pinning events (out of 400 injected domain walls for each field), for a 1.4 V–10 ns injection pulse (red curve in a ). The black dashed line shows how the drop of the pinning probability in the red curve on a , corresponds with the disappearance of the low-resistive domain walls (Transversal domain wall). Note that the colour scale on the right is not linear. Full size image Now, we focus on the increase of the pinning probability for higher fields. Figure 3a shows that, for fields higher than 3 Oe, the probability of pinning rises gradually until it plateaus just over 0.2 for fields larger than 10 Oe. The probability drops again for fields larger than 35 Oe until it reaches zero after 50 Oe. As mentioned above, the type of DW nucleated in our experiments is always transversal (Δ R =0.19 Ω). On the other hand, as it can be seen in Figure 3b , after 3 Oe, the pinning events distribute between VW (Δ R =0.29 Ω) and transversal DW (Δ R =0.23 Ω). Also the resistance of the TW increases slightly as the field increases, indicating that its shape is slightly different for the pining events at higher fields. Additionally at 35 Oe, where the pinning probability starts to drop, the transversal DW is never found among the pinning events, leaving only increasingly resistive DW, as the magnetic field gets larger. The regions of pinning just described match well with the different DW propagation modes: translational mode up to the Walker breakdown (around 10 Oe for this type of stripes), precessional mode up to about 20–30 Oe and a turbulent mode for higher fields. These field values were obtained from previous simulations [9] and match well with other experimental reports in permalloy nanostripes of the same [1] , [12] or even different dimensions [13] , [14] . In the translational mode, the structure of the DW is stable during its displacement. In our case, as the nucleated DW is always transversal, it should travel, keeping its transversal structure for very low fields. In the precessional mode, for fields larger than about 10 Oe, the DW undergoes periodic transformations, from TW to VW [15] , [16] . Finally, in the turbulent mode [17] , vortex and antivortex DW are nucleated in the stripe and at the edges, undergoing gyrotropic motions and annihilations as they travel. The type of DW wall that gets pinned at each field ( Fig. 3b ) matches well with these different modes. As the field approaches 10 Oe, both types of DWs get pinned as both are present in the precessional mode. Interestingly, after 10 Oe, the pinning probability stays constant with the field and both types of DWs are found in the pinning events. This again agrees with having a precessional mode in the DW motion as the average DW velocity changes very little with the external field during this regime [16] . Finally, for larger fields (over 35 Oe), the only pinning events have quite a large resistance (Δ R >0.32 Ω), which indicates that only very wide and stretched DWs have a chance of being pinned at such a large magnetic field, in concordance with the DW being in a turbulent regime. The fact that the probability of pinning follows the propagation regimes of the DW, indicates that the pinning is intrinsic to the DW motion on magnetic nanostripes and therefore, quite possibly, unavoidable in real (not simulated) structures except for very low fields, as we have shown. We still have to find out the influence of the Oersted field created by the injection pulse in our results. Although the in-plane Oersted field from the current pulse is negligible further than 500 nm away from the current line, the perpendicular to plane field reaches considerable values along the entire length of the magnetic stripe. For the current density of 1 V pulse (1.45×10 8 Acm −2 ), the perpendicular to plane field is about 400 Oe by the edge of the current line, ∼ 40 Oe 2 μm away and ∼ 20 Oe 4 μm away from the current line [18] . Therefore, this field is not negligible and its influence has to be evaluated. 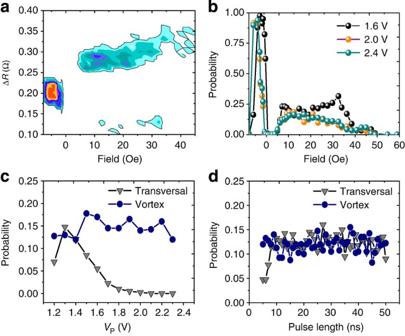Figure 4: Enhanced pinning in the precessional mode and the pinning probability for different types of magnetic domain wall. (a) Resistance map showing the pinning events for a 25 ns–2 V injection pulse, versus the applied field. The colour code is the same as that inFigure 3b. (b) Probability of pinning (0–1) for a 25 ns injection pulse and different amplitudes. (c) Probability of pinning (0–1) for the different types of domain wall versus the amplitude of the pulse at a fixed field of 12.5 Oe and for a 25 ns injection pulse. (d) Probability of pinning (0–1) for both types of domain wall versus the pulse length, for a pulse amplitude of 1.4 V and an external field of 12.5 Oe. Figure 4a shows a map with the resistance of the pinning events for a 25 ns–2 V injection pulse. As it can be seen the TWs are absent from the pinning events for fields larger than 3 Oe. The pinning probability versus the applied magnetic field for a 25 ns pulse and several pulse amplitudes is shown in Figure 4b . In the 10–30 Oe field range, at low-pulse amplitudes, the probability plateaus over 0.2 (like in the results shown in Fig. 3a ) whereas, for higher pulse amplitudes, it gradually decreases after 10 Oe. Interestingly, Figure 4c also shows that although the probability of pinning a VW is not affected by the pulse amplitude, the probability of pinning a TW drops quickly to zero as the pulse amplitude is increased. It has been shown using micromagnetic simulations that a perpendicular to plane magnetic field can stabilize the TW structure and even suppress the Walker breakdown [19] . In our experiments, at low pulse amplitudes (that is, small field perpendicular to plane) and intermediate fields (10–35 Oe), the probability of pinning is the same for both types of DW for any pulse length ( Fig. 4d ), although the TW disappears from the pinning events as the amplitude is increased ( Fig. 4c ). As the TW is present in section AB of the nanostripe for all pulse amplitudes ( Fig. 2c–e ), the perpendicular to plane field from the injection pulse might be enhancing the transmission probability for the TW. This was also shown in ref. 9 , where the simulations showed that, on a finite-length stripe, the perpendicular to plane field from the current line, promotes the TW after nucleation. It is interesting that, in the precessional mode, the DW is in the vortex configuration for longer periods of time than in the transversal configuration (although the velocity is larger while being transversal) [16] , but their pinning probabilities are the same ( Fig. 4d ). Figure 4: Enhanced pinning in the precessional mode and the pinning probability for different types of magnetic domain wall. ( a ) Resistance map showing the pinning events for a 25 ns–2 V injection pulse, versus the applied field. The colour code is the same as that in Figure 3b . ( b ) Probability of pinning (0–1) for a 25 ns injection pulse and different amplitudes. ( c ) Probability of pinning (0–1) for the different types of domain wall versus the amplitude of the pulse at a fixed field of 12.5 Oe and for a 25 ns injection pulse. ( d ) Probability of pinning (0–1) for both types of domain wall versus the pulse length, for a pulse amplitude of 1.4 V and an external field of 12.5 Oe. Full size image The perpendicular to plane field from the current pulse could also affect the DW motion in the low field range, when the pinning probability is zero. The velocity of a DW in these type of nanostripes at low fields has been measured many times by different groups and it should be smaller than 100 m s −1 . In this case, for pulses shorter than 25 ns (and very low fields), the DW should still be travelling through the nanostripe when the pulse finishes. Therefore, the Oersted field from the injection pulse may trigger the initial movement of the DW but cannot justify its perfect transmission probability at very low fields, which must be a consequence of the rigid structure of the DW, when moving at very small velocity (low field regime). We have shown that the stochastic pinning of a DW in magnetic nanostripes follows different field regimes that match the propagation modes of the DW. This stochastic behaviour of the DW can be suppressed for very low fields, where the structure to the DW should not suffer any viscous transformations or deformations. In this regime, the DW can be transmitted reliably without ever pinning. At very low fields, the velocity and the kinetic energy of the DW are very small, and it might seem counterintuitive to find that it is precisely in this regime where the DW never gets pinned along the stripe. In fact, other results have shown that the depinning of a DW from a notch is more efficient when the DW is moving (kinetic field depinning smaller than static field depinning) [20] , [21] . These results are measured for strong pinning potentials (notch or anti-notch) whereas our results are measured in the weak pinning regime. In this weak pinning regime, the probability of pinning increases for higher fields (higher speed), quite likely due to the relation between the phase of the DW and the local potential [4] . In this low pinning regime, as soon as the external field provides enough energy for the DW to achieve shape transformations or deformations, there is an increasing chance for the DW to adapt to the local microstructure and to minimize its energy by getting pinned. The pinning probability increases gradually from very low fields ( ∼ 3 Oe) until it plateaus around 10 Oe (approximately the Walker breakdown field in permalloy stripes of these dimensions). This means that, even for fields considerably smaller than the Walker breakdown (the beginning of the precessional regime), there is a non-zero probability of finding outlying events, where the DW travels in the precessional mode even for fields well within the translational mode. We are aware that the enhanced DW pinning at high fields has been observed before [4] , [7] . The results from refs 4 and 7 indicated also that the probability of pinning at low fields could be quite low. Our results, in contrast, show distinctively that this probability of pinning follows the same modes than the DW motion and provide evidence that it can be completely suppressed at very low fields. This work highlights the necessity of designing the racetrack devices with materials and geometries that can delay the Walker breakdown to higher fields [22] , [23] . Additionally, a perpendicular-to-plane field seems to enhance the transmission probability. This could be implemented easily on a race-track device by depositing a hard magnetic material as a buffer layer with the magnetization perpendicular to plane. Sample preparation and device fabrication The nanostripes were fabricated by DC magnetron sputtering and lift-off on Si/SiO 2 , substrates with the structure Cr (1 nm) per Ni 80 Fe 20 (10 nm) per Au (0.5 nm). The contacts and current line were also DC-sputtered with the structure Cr (1 nm) per Au (60 nm). The surface of the sample was passivated after fabrication to avoid deterioration and oxidation with time. Measuring procedure Each event is constituted by the following sequence: the nanostripe was saturated with 1,500 Oe in the negative direction ( Fig. 1a ) and then the applied field is set before the injection pulse is applied. There is a 2-s integration time to measure the drop of the resistance caused by the DW before starting the next event. The pulse rise time is 1.9 ns, measured on a digital oscilloscope connected between the exit of the current line and ground (channel impedance is 50 Ω). For pulse amplitudes below 1 V, the DW is not injected and, for pulses over 2.4 V, there is a good chance of destroying the device. How to cite this article: Muñoz, M. et al . Suppression of the intrinsic stochastic pinning of domain walls in magnetic nanostripes. Nat. Commun. 2:562 doi: 10.1038/ncomms1575 (2011).